Discovery of extended product structural space of the fungal dioxygenase AsqJ 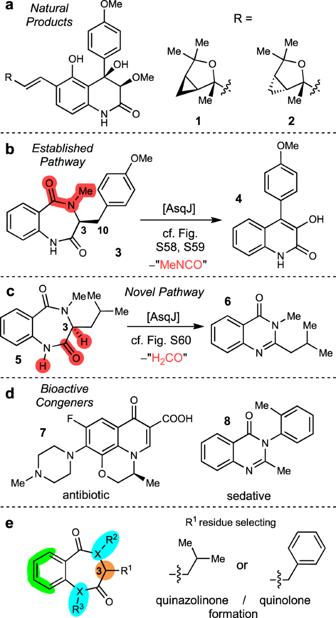Fig. 1: Relevance and substrate promiscuity of AsqJ. aStructures of the natural products aspoquinolones A (1) and B (2).bBiosynthetic transformation of3to quinolone4catalysed by AsqJ.cPathway of AsqJ from5to quinazolinones6. The molecular portions labelled in red get excised in the course of the AsqJ catalytic transformation.dExamples of drugs with quinolone and quinazolinone motifs: levofloxacin (7) and methaqualone (8).eGraphical summary of AsqJ substrate structural alterations evaluated in this study across the quinazolinone (R1=iso-butyl) and quinolone (R1= benzyl) pathways. The fungal dioxygenase AsqJ catalyses the conversion of benzo[1,4]diazepine-2,5-diones into quinolone antibiotics. A second, alternative reaction pathway leads to a different biomedically important product class, the quinazolinones. Within this work, we explore the catalytic promiscuity of AsqJ by screening its activity across a broad range of functionalized substrates made accessible by solid-/liquid-phase peptide synthetic routes. These systematic investigations map the substrate tolerance of AsqJ within its two established pathways, revealing significant promiscuity, especially in the quinolone pathway. Most importantly, two further reactivities leading to new AsqJ product classes are discovered, thus significantly expanding the structural space accessible by this biosynthetic enzyme. Switching AsqJ product selectivity is achieved by subtle structural changes on the substrate, revealing a remarkable substrate-controlled product selectivity in enzyme catalysis. Our work paves the way for the biocatalytic synthesis of diverse biomedically important heterocyclic structural frameworks. The Fe II /α-ketoglutarate-dependent fungal dioxygenase AsqJ from Aspergillus nidulans was discovered in 2014 by Watanabe et al. [1] and characterised as a key enzyme in the biosynthesis of fungal alkaloids, such as the aspoquinolones A and B ( 1 and 2 , Fig. 1a ) [2] , [3] , [4] . The non-heme enzyme catalyses a fascinating reaction cascade, involving a one-pot desaturation/epoxidation reaction of a N 4 -methylated benzo[1,4]diazepine-2,5-dione 3 with concomitant ring-contraction/fragmentation to the viridicatin scaffold ( 4 , Fig. 1b ; for detailed mechanism, see Figs. S58 and S59 ). The single steps of this reaction cascade, as well as the function of other enzymes in the viridicatin biosynthetic gene cluster, were described in detail by different research groups [3] , [5] , [6] , [7] , [8] , [9] . In our recent study, we discovered an unprecedented additional reactivity of this enzyme [10] . While substrates with a methylene-bridged aryl substituent at C 3 -position of the 7-membered substrate core were converted to quinolin-2(1 H )-ones, most of the other tested substrates were transformed into quinazolin-4(3 H )-ones, for example 5 to 6 , thereby following a new enzymatic pathway, involving α-lactam formation, hydrolysis and oxidative decarboxylation (Fig. 1c , for detailed mechanism, see Fig. S60 ). Fig. 1: Relevance and substrate promiscuity of AsqJ. a Structures of the natural products aspoquinolones A ( 1 ) and B ( 2 ). b Biosynthetic transformation of 3 to quinolone 4 catalysed by AsqJ. c Pathway of AsqJ from 5 to quinazolinones 6 . The molecular portions labelled in red get excised in the course of the AsqJ catalytic transformation. d Examples of drugs with quinolone and quinazolinone motifs: levofloxacin ( 7 ) and methaqualone ( 8 ). e Graphical summary of AsqJ substrate structural alterations evaluated in this study across the quinazolinone (R 1 = iso -butyl) and quinolone (R 1 = benzyl) pathways. Full size image Both heterocyclic product classes accessible by AsqJ are of exceptional biomedical relevance, as exemplified by the drugs levofloxacin (quinoline-4(1 H )-one 7 ) and methaqualone (quinazolinone 8 ), which possess antibacterial and strongly sedative activities, respectively. Within this study we set out to systematically evaluate the promiscuity of AsqJ, thereby not only systematically mapping its biocatalytic flexibility, but also aiming at the discovery of potential further reaction trajectories towards other biomedically relevant heterocycles. This indeed led to the discovery of further product classes addressable by AsqJ, significantly expanding AsqJ product structural space. Given our recent findings on product selectivity of AsqJ [10] , which revealed highly selective and efficient transformations of iso -butyl or benzyl R 1 -substituted substrates to quinazolinones and quinolones, respectively, we selected these two substitution patterns as main templates for the investigation of AsqJ substrate structure tolerance across its bimodal biocatalytic activity (Fig. 1e ). These substrates were systematically altered with respect to substitution at the aromatic ring (green), configuration at the stereogenic center at C 3 (orange), as well as the nature of the heteroatom X (nitrogen or oxygen) and, for N -containing substrates, the substitution pattern at R 2 /R 3 (blue). In addition, tricyclic congeners in which R 1 and R 2 are connected within a five- or six-membered ring system were evaluated. Investigation of aromatic core substitution The investigations were initiated by testing the promiscuity of AsqJ towards substitutions at the western aromatic core, which is unsubstituted in all natural substrates. The modifications were introduced by employing substituted anthranilic acid building blocks to enable an expedited production of diversely functionalized substrates. Since N 4 -methylation of the substrate was shown to be necessary for enzymatic transformation in previous studies [5] , [6] , [10] , our solid phase peptide synthesis (SPPS)-based approach to benzo[1,4]diazepine-2,5-diones 9 / 10 was refined by loading already N α -methylated amino acids 11 onto Wang resin. These were easily accessible by a two-step sequence from commercially available Fmoc-protected amino acids 12 , by oxazolidinone 13 formation and subsequent reductive cleavage to 11 (see SI, chapter 2.1.1 for individual yields) [11] . After loading 11 onto Wang resin under Steglich conditions to deliver 14 , Fmoc deprotection with piperidine gave secondary amines 15 . These were coupled to Fmoc-protected acids 16 that were synthesised from commercially available substituted anthranilic acids 17 (see SI, chapter 2.1.2 for individual yields), including fluoro- ( 17a–d ), chloro- ( 17e–g ), nitro- ( 17h ) and methyl- ( 17i–k ) substituents, as well as naphthoic acid 17l . Couplings proceeded smoothly with HATU, HOAt and DIPEA in DMF to deliver dipeptides 18 . These were deprotected with piperidine to yield free amines 19 . Sodium tert -butoxide-induced cyclization with concomitant off-loading from the resin gave the desired compounds 9 / 10 . In case of the nitro substituted analogues 9h / 10h , these cyclization conditions led to decomposition. As the 7-membered ring can also be formed by an acid-induced cyclization [10] , [12] , we alternatively employed 35% TFA in DCM for the synthesis of 9h / 10h , leading to the desired cyclization with concomitant cleavage from the Wang resin (Fig. 2a ). Taken together, 24 substrates with modifications at their aromatic core were synthesised (Fig. 2b ; see SI for further details regarding yields of intermediates etc.) and hence available for AsqJ promiscuity studies. Fig. 2: Combinatorial substrate synthesis by SPPS. a Synthetic route towards N 4 -methylated benzo[1,4]diazepine-2,5-diones with different substitutions at the aromatic core, as indicated in blue. b Overall yields of the respective products 9/10 from 14 (over four steps). DCM dichloromethane, DIC N , N ’-diisopropylcarbodiimide, DIPEA N , N -diisopropylethylamine, DMAP 4-dimethylaminopyridine, DMF N , N -dimethylformamide, FG functional group, Fmoc fluorenylmethyloxycarbonyl, HATU hexafluorophosphate azabenzotriazole tetramethyl uronium, HOAt 1-hydroxy-7-azabenzotriazole, TFA trifluoroacetic acid, THF tetrahydrofuran. Full size image AsqJ substrate promiscuity was evaluated with recombinantly produced enzyme and an LC-MS-based activity assay (see SI, chapters 1.2 and 3.1 for details) [5] , [10] . To allow the comparison of transformations for different substrates, the assays were quenched at a maximum of 8 hours by TFA addition, even if substrate conversion was incomplete. For the pathway to quinazolinones, only fluorinated compounds 9a to 9d were accepted by the enzyme with clearly detectable product formation. To gain deeper insights into these conversions, we scaled up the corresponding assay with substrate 9c and isolated all (side-)products by preparative HPLC. Beside the expected quinazolinone 21c , putatively formed via 20c , a more polar compound was also obtained (Fig. 3a , top). 1 H NMR showed that the iso -butyl residue in this additional product was absent, indicating that substrates entering the quinazolinone pathway can also be transformed by excision of the corresponding former amino acid side chain. This would result in formation of a quinazoline-2,4(1 H ,3 H )-dione 22c . While comparison of the analytical data with NMR data from the literature already strengthened this assumption [13] , chemical synthesis (cf. ESI, chapter 2.3) and overlay of 1 H NMR spectra (cf. ESI, Fig. S245 ) unambiguously corroborated the structure of 22c . This additional product was also detected for other substrates following the quinazolinone pathway. To further investigate the unknown mechanism of formation of this new product class, we incubated chemically synthesised 6 [10] (cf. Fig. 1c ) with AsqJ to evaluate if side-chain cleavage occurs as the last step in quinazolindione formation. No conversion was observed (cf. Fig. S2 ), hence pointing towards a synchronous rather than a sequential formation of the quinazolindione. To corroborate this proposal, conversion of 1- 13 C-alanine-derived substrate [10] ( 23 ) was conducted and investigated by HRMS and NMR. In contrast to the formed quinazolinone ( 24 ), the corresponding quinazolindione ( 25 ) had the labelled carbon still present (see Fig. 3b ; and SI, chapter 3.3 for details), thus clearly showing that compound class 22 is directly formed from substrate 9c in an alternative reaction pathway (see Fig. S61 for detailed proposals on the new mechanism). This establishes quinazolindiones such as 22 as an additional heterocyclic compound class being accessible by AsqJ. The enzyme catalyses a ring contraction reaction with concomitant cleavage of the aliphatic side-chain at C 3 . This is an important finding, as the resulting product core structure is of considerable biomedical interest, as exemplified by the aldose reductase inhibitor Zenarestat (FK-366, 26 ) [14] or 5-hydroxytryptamine 5A (5-HT 5A ) receptor antagonist KKHT10612 [15] ( 27 , Fig. 3a , bottom). Fig. 3: AsqJ assay results for selected substrates. a Summary of substrate screening outcomes for the quinazolin(di)one pathway (exemplarily shown for 9c ) and structures of quinazolindione biomedical agents 26 and 27 . b Difference in ring contraction for quinazolinone and quinazolindione products as observed by conversion of 13 C-labelled substrate 23 . c Summary of substrate screening outcomes for the quinolone pathway (exemplarily shown for 10b ). HT hydroxytryptamine. Full size image For the well-established pathway towards quinolones 28 , AsqJ showed very broad promiscuity towards all substituted substrate analogues, except naphthyl-based 10l . Especially for the fluorinated and methylated compounds 10a–d and 10i–k , a high up to complete conversion to desaturated ( 29 ) and epoxidized ( 30 ) intermediates was observed (Fig. 3c , exemplarily shown for 10b ). Interestingly, the final fragmentation reaction to the corresponding quinolones 28 showed dependency on the aromatic substituent. For example, the assay with 7-Me-substituted substrate 10j showed nearly complete conversion to quinolone 28j , whereas 8-nitro compound 10h was only converted to its epoxide 30h . This observation can possibly be explained by the electronic effects of the corresponding substituents (σ + vs . π – ), hence accelerating or inhibiting the nucleophilic attack of the western aromatic ring on the strained epoxide that results in formation of the final product (cf. Fig. S59 ). It is interesting to note that it appears that the rearrangement reaction from epoxides 30 to quinolones 28 is significantly accelerated by an acidic environment. To probe this, we repeated assays with 10c and 10j on a mg scale and monitored progress of the reaction after 90 minutes by HPLC, once after quenching by addition of TFA, once by acetonitrile (ACN) addition. The chromatograms of the assay with fluorinated compound 10c showed the presence of desaturated ( 29c ) and epoxidized ( 30c ) substrate, but no formation of quinolone 28c for both quenching methods. In contrast, the chromatogram of the assay with methylated substrate 10j showed formation of small amounts of the final product 28j after quenching with TFA, but not for ACN quenching (see Fig. S46 ). The observed difference between the substrates may result from the different substituents at the western aromatic portion, hence altered electronic effects during the fragmentation reaction (as described above). The finding that acidic reaction conditions accelerate the rearrangement from epoxide 30 to quinolone 28 goes in hand with a recent study by Chang et al., who induced the ring-contraction by addition of the Lewis acid BF 3 •OEt 2 [16] . It also explains the presence of a dedicated additional enzyme in the biosynthetic pathway of viridicatin scaffolds, AsqI, assisting the final rearrangement reaction under physiological conditions, as recently shown by Kishimoto et al. [2] . To further investigate the influence of reaction conditions on the final fragmentation reaction from epoxides 30 to quinolones 28 , we performed upscaled AsqJ assays with substrate 10d . After workup by extraction with DCM, 16 different defined conditions were tested, including variations of solvent (acetone vs . chloroform vs . methanol vs . tetrahydrofuran), reaction temperatures (22 °C vs . 50 °C) and acidic reagents (TFA vs . BF 3 •OEt 2 ). Interestingly, most of these experiments only delivered minute amounts of the desired product 28 . For most reaction conditions, formation of a more polar side-product was observed, most prominently in CHCl 3 at 50 °C using TFA. HRMS analysis indicated this compound to represent 1,2-diol 31d , originating from acid-induced activation of the epoxide followed by its nucleophilic opening by water. In methanol, the reactivity of the epoxide was strongly decreased, as little to no turnover was observed when compared to the untreated starting material. Most importantly, however, these investigations revealed that conducting the reaction in CHCl 3 with BF 3 •OEt 2 at room temperature facilitates complete and selective conversion of 30d to the desired quinolone 28d (cf. Figs. S47 and S48 for details). Taken together, while TFA seems to accelerate the fragmentation reaction under aqueous (assay) conditions, BF 3 •OEt 2 is the method of choice in organic solvent, with CHCl 3 at room temperature delivering best results in terms of both, conversion and selectivity. Another interesting observation was made in the case of methyl substituted substrates 10i, 10j and 10k , where — among the respective expected products 30 and 28 — the corresponding quinazolinones 32i, j, k were also present in the assay mixture, yet in small amounts. Quinazolinone formation apparently occurs as an alternative reaction path in these cases, since these compounds are less suitable for the natural reaction trajectory. Evaluation of the impact of C 3 -configuration In addition to all natural AsqJ substrates and all other analogues tested within this study that are derived from l -amino acids and thus are ( S )-configured, we set out to investigate the enzymatic transformation with ( R )-configured substrates. A previous study described that the AsqJ-catalysed reaction proceeds irrespective of the C 3 -configuration of the substrate [8] . To corroborate these findings and furthermore test the effect of altered C 3 -configuration on the AsqJ pathway leading to quinazolinones, the ( R )-configured substrates, ( R )- 9 and ( R )- 10 , were also synthesised following a previously established SPPS route [10] by using the respective Fmoc-protected d -amino acids ( R )- 12 as starting materials (see SI for experimental details). The assays with these epimerized substrates delivered interesting findings: in the case of C 3 -epimerized ( R )- 10 complete consumption was observed in accordance with earlier investigations [8] . This goes in hand with the mechanistic proposal that the quinolone reaction pathway starts with radical formation at C 10 , followed by formation of a carbocation or a hydroxylated intermediate [7] . As a consequence, C 3 -epimerization does not affect the corresponding reaction mechanism. The assay with ( R )- 9 , however, showed only very poor conversion. In contrast to the quinolone pathway, quinazolin(di)one formation is supposed to commence with a homolytic hydrogen abstraction at C 3 -position [10] . Epimerization of the C 3 -stereocenter hence has a direct effect on this initial radical formation and appears to strongly inhibit this reactivity (see Fig. 4 ). The minimal turnover still observed is rather a consequence of minute epimerization of the substrate ( R )- 9 under assay conditions or during substrate synthesis (in particular base-induced cyclization/off-loading reaction with NaO t Bu, cf. Fig. 2a ) followed by transformation of the minute amounts of ( S )- 9 thus available to AsqJ. It is interesting to note that assays with ( R )- 10 showed formation of an additional product by HPLC analysis. While isolation was successful, unambiguous characterization based on 1 H NMR alone did not allow characterization and further NMR analysis was not possible due to very low isolated product amounts. Fig. 4: Investigations of substrate stereochemical influence. Results of enzyme assays with ( R )-enantiomers of 9 and 10 and supposed explanation. Full size image Taken together, it can thus be stated that C 3 -epimerization is unfavourable for both pathways, either in terms of selectivity (quinolone pathway) or efficiency (quinazolin(di)one pathway) of the enzymatic transformation. Exploring the effects of N -substitution at the central 7-membered ring Given the requirement of AsqJ for an N 4 -methylated substrate for successful enzymatic conversion, investigations into its promiscuity towards other N 4 -alkyl functions were also targeted. Therefore, synthesis of compounds 9m and 10m , as well as two additional substrates 33 and 34 derived from cyclohexylalanine and ( O Me)-tyrosine, respectively, carrying an N 4 -ethyl substituent was carried out, initially following the established SPPS approach (see SI for details). After the first synthetic steps, including N -ethylation under Mitsunobu conditions [17] , which yielded the N α -ethylated amino acids 35 , the coupling step with Fmoc-aminobenzoic acid ( 16 ) failed under all tested conditions (Fig. 5 ). Even very potent coupling reagents, such as PyBroP or DFIH (1,3-dimethyl-2-fluoro-4,5-dihydro-1 H -imidazolium hexafluorophosphate), did not yield the desired coupling products 36 , likely due to the increased steric hindrance caused by the N -ethyl group. As a workaround, the coupling was conducted with 2-nitrobenzoic acid ( 37 ) [18] , since the nitro group exhibits less steric demand during the coupling reaction and additionally increases the acidity of the benzoic acid. Subsequent reduction of the nitro compounds 38 to the corresponding amines 39 using 2 m tin(II) chloride in DMF and cyclization as described above delivered the desired N 4 -ethylated substrates (see Fig. 5 for individual yields) [18] . Fig. 5: Optimized synthesis of N 4 -ethylated substrates [18] . Yields are given over seven steps, starting from loaded resin. DFIH 1,3-dimethyl-2-fluoro-4,5-dihydro-1 H -imidazolium hexafluorophosphate, PyBroP bromotripyrrolidinophosphonium hexafluorophosphate. Full size image During purification of the cyclized N 4 -ethylated compound 10m derived of phenylalanine, we discovered a second compound with slightly lower retention time on RP-HPLC, hence increased polarity. Isolation and HRMS/NMR analyses revealed this to be N 1 -hydroxylated compound 40 , which results from incomplete reduction of the aromatic nitro group to hydroxylamine 41 and subsequent base-induced cyclization. This unexpected side-reaction paved the way for the additional evaluation of this N -hydroxylated substrate analogue 40 . Interestingly, all N 4 -ethylated compounds were accepted and converted by AsqJ (Fig. 6 ). Enzyme reactions with 9m and 32 proceeded following the quinazolinone pathway to N 3 -ethylated quinazolinones 42 and 43 (with observation of presumed corresponding quinazolin-2,4-dione 44 , and desaturated side-product 45 ), while 10m and 34 were converted following the quinolone mechanism with concomitant elimination of ethyl isocyanate. The N 1 -hydroxylated compound 40 was accepted as a substrate, but conversion stopped at the stage of the epoxide 46 via desaturated compound 47 , comparable to the nitro compound 10h . This observation fits to the mechanistic proposal that an abstractable hydrogen at the N 1 atom facilitates the fragmentation reaction [5] . Fig. 6: AsqJ assay results with N 4 -ethyl analogues. a Biocatalytic transformation of N 4 -ethylated substrates. b Conversion of the additionally N 1 -hydroxylated analogue 40 , where no quinolone formation was observed. Cy cyclohexyl, An 4-anisolyl ( p -methoxyphenyl). Full size image In addition to N 4 -alkylation, the effect of N 1 -methylation on AsqJ catalysis was explored. Optimization of a test reaction with commercially available glycine-derived benzo[1,4]diazepine-2,5-dione 48 yielded the dimethylated compound 49n in 38% yield by deprotonation with sodium hydride followed by treatment with methyl iodide in THF. Following this approach, compounds 9 and 10 were converted to their double methylated congeners 9n and 10n in 67% and 78%, respectively (Fig. 7a ). Fig. 7: Synthesis and conversion of N , N -dimethylated substrates. a Late-stage methylation (blue) towards the desired compounds. b Results of enzymatic conversion with mechanism proposal for hydroxylation of 49n (proposed origin of hydroxyl group labelled in green), as well as structure of blockbuster pharmaceutical lorazepam ( 51 ). Full size image Enzymatic conversion of the N 1 -methylated substrate 49n (in which R = H) led to formation of a single product (Fig. 7b ). Upscaling and isolation allowed investigation of its structure by 1 H NMR and HRMS, which showed that the C 3 -hydroxylated compound 50 was formed. This defines yet another reactivity accessible by AsqJ catalysis, leading to a product that has structural similarity to the blockbuster pharmaceutical lorazepam ( 51 ). We assume that the N 1 -methyl group blocks the N 1 – C 3 bond formation of the quinazolinone pathway, hence leading to an intermediate free carbon-centred radical or carbocation I1 (after a second radical abstraction, cf. Fig. S61 ) at C 3 , which is ultimately trapped by water (free or enzyme-bound). To mechanistically investigate whether this is an enzymatic or non-enzymatic process, stereochemical analysis of 50 was of high interest. While an enantiopure or -enriched product would hint towards an enzymatic hydroxylation, a racemic mixture would rather point towards non-enzymatic capture of an intermediate radical or ion ( I1 ) by a water molecule. It has to be taken into account, however, that 3-hydroxylated diazepines such as 50 are highly prone to epimerization. For example, enantiopure lorazepam ( 51 ) was shown to have a half-live time of about 21 minutes [19] . We therefore investigated the optical purity of freshly prepared 50 by rapid analysis by HPLC on a chiral phase. These investigations revealed 50 to occur as racemic mixture, pointing at a non-enzymatic quenching reaction or very fast loss of stereochemical integrity due to racemization (cf. ESI, chapter 3.3; Fig. S44 ). To further distinguish between these possibilities, we performed an enzyme assay with substrate 49n and H 2 18 O as reaction solvent (approx. 80 vol-%). By HRMS, we observed that approx. 36% of 50 were indeed 18 O-labelled, as indicated by the corresponding mass counts (cf. ESI, Fig. S45 ). These results further substantiate the hypothesis that the hydroxyl group originates from water quenching of an enzyme-activated intermediate, such as I1 (Fig. 7b ). For the N 1 -methylated substrate 9n , the assay showed only trace consumption of substrate with formation of unidentified products in minute amounts. In the case of 10n , epoxidized compound 30n was observed, as well as a small amount of fragmentation product 28n . Moreover, an additional, large product peak was detected by HPLC analysis. Up-scaling of the reaction and isolation of this compound was attempted to facilitate downstream NMR and HRMS analyses. However, its characterization was not possible due to product instability. Taken together, it can be stated that N 1 -substitution is not favourable for either the quinazolinone or the quinolone pathway, yet paves the way for a new biocatalytic aliphatic C -hydroxylation in glycine-derived substrate analogue 49n . AsqJ biocatalytic fidelity towards tricyclic substrates As a further expansion of the possible substrate scope, we produced compounds in which the R 1 and R 2 residues are part of a five- or six-membered cyclic ring system, synthetically derived from proline ( 52 ) or pipecolic acid ( 53 ), respectively. The synthesis was accomplished in 44% ( 54 ) and 83% ( 55 ) following the solid-phase peptide synthesis (SPPS) approach described earlier (Fig. 8a ) [10] . This resulted in a very fast synthetic access to this compound class by loading of the Wang resin to give esters 56 / 57 , Fmoc deprotection to secondary amines 58 / 59 , coupling with 16 to the dipeptides 60 / 61 , second deprotection to aromatic amines 62 / 63 and base-induced cyclization to 54 / 55 . To our delight, although with overall lower turnover (cf. quantification of the transformation of key substrates below), enzymatic conversion of tricyclic substrate 54 proceeded to give tricyclic quinazolinone natural product deoxyvasicinone ( 64 , Fig. 8b ), a compound reported to be found in, e.g., Peganum harmala L. seeds [20] . This result emphasizes the versatility of AsqJ, underlining its potential use in chemo-enzymatic natural product synthesis. Interestingly, compound 64 represents the carbon scaffold of the plant-derived natural products vasicinone ( 65 ) from Adhatoda vasica Nees [21] and its regioisomer isovasicinone ( 66 ). 65 and 66 show antifungal activity against, e.g., Fusarium graminearum and Helminthosporium sativum [22] . To further proof the applicability of AsqJ in bioactive natural product synthesis, we aimed at the chemo-enzymatic synthesis of isovasicinone ( 66 ). Starting with hydroxyproline 67 , Fmoc- and TBS-protection at the amine and hydroxy functionalities delivered building block 68 (cf. ESI 2.1.2), which was incorporated into hydroxylated precursor 69 (cf. ESI 2.2.1) (Fig. 8d , top). Fig. 8: Investigations involving tricyclic substrates. a Synthesis of tricyclic substrates 54 / 55 . b Enzymatic conversion. c Synthesis of hypothesized aldehyde 76 and comparison with isolated compound 74 . Green colour indicates same chemical formulas and hence m/z ratios of these compounds. d Synthesis and conversion of l -4-hydroxyproline-derived substrate 69 . NMR nuclear magnetic resonance, TBS tert -butyldimethylsilyl. Full size image AsqJ assays with this substrate indeed led to formation of the desired antifungal compound isovasicinone ( 66 ). In addition, a small amount of side-product was observed. Isolation and NMR characterization was not possible because of the very small amounts produced, but HRMS indicated a loss of hydrogen and water when compared to 69 . We therefore propose this compound to be pyrrole 70 , whose formation can be explained by initial AsqJ-catalysed dehydration of 69 to 71 followed by elimination of the secondary alcohol to deliver the aromatic system (Fig. 8d ). Application of l -pipecolic acid-derived substrate 55 led to formation of quinazolinone 72 , representing the natural product mackinazolinone isolated from Mackinlaya sp [23] . In addition to 72 , formation of desaturated side-product 73 was observed. Moreover, both assays showed formation of an additional, more polar side-product. Unambiguous structure elucidation after attempted isolation of this side-product in the conversion of 54 was not possible due to the minute amounts formed, but 1 H-NMR and HRMS indicated this substance to be the intermediate acid ( 74 and analogously 75 ) of the quinazolinone pathway. As potential alternatives to formation of side-product structures 74 / 75 , the above described, newly discovered side-chain excision mechanisms for bicyclic substrates leading to quinazolindiones, e.g., 22c (cf. Fig. 3a/b ) were also considered. With tricyclic substrates, this reaction would potentially lead to ring opening of the five- ( 54 ) or six- ( 55 ) membered eastern ring originating from the cyclic amino acids 52 / 53 . Following our mechanistic proposal for the quinazolindione pathway (cf. Fig. S61 ), in the case of 54 this would furnish the bicyclic aldehyde 76 (cf. Fig. 8c ). As the molecular masses of the proposed acid intermediate 74 compared to the resulting, hypothetical 76 would be identical, we desired to experimentally test this alternative hypothesis. Therefore, we conducted the synthesis of aldehyde 76 in a five-step route starting from isatoic anhydride ( 77 ) and 4-aminobutanol ( 78 ) in an overall yield of 31% (cf. ESI, chapter 2.3 for experimental details). Comparison of the spectroscopic data ( 1 H NMR) of the observed side-product compared to synthetic aldehyde 76 showed no match (cf. Fig. S246 ), hence further substantiating this compound to indeed correspond to acid 74 . Probing the exchange of the nitrogen (amide) by oxygen (ester) heteroatoms Moreover, replacement of the amide moieties in 9/10 as esters to generate oxygen-containing heterocyclic compounds by enzymatic conversion using AsqJ deemed interesting to us. For the northern substitution (towards 79 ), we developed a short reaction sequence starting from lactic acids 80 (Fig. 9a ). After methyl ester protection with thionyl chloride to 81 , esterification with 2-nitrobenzoic acid ( 37 ) under Steglich conditions delivered esters 82 . After saponification with KOH to the free acids 83 with short reaction time to avoid cleavage of the desired ester, and Pd-assisted hydrogenation of the nitro group to amino acids 84 , HATU-mediated cyclization afforded cyclic amides 79 (see Fig. 9a for individual yields). For the southern esters ( 85 ), resin-bound N -methylated amino acids ( 15 ) were coupled to salicylic acid ( 86 ) under standard conditions (HATU, HOAt, DIPEA) in a reduced amount of time to avoid undesired esterifications, affording phenols 87 . Unfortunately, base-induced cyclization of 87 was unsuccessful with the alcohol instead of the amine. Cleavage from the resin with 35% TFA in DCM to the corresponding hydroxy acids 88 before HATU-assisted cyclization delivered the desired products 85 (see Fig. 9b for individual yields). However, these esters were unstable during purification, presumably because of the conjugated acid motif, imparting reactivity of vinylogous anhydrides (cf. Fig. 9c , labelled in yellow). Therefore, these substances were subjected to AsqJ directly after workup without further purification. Fig. 9: Syntheses and assays of ester substrate analogues. a Route to benzo[ e ]oxazepines 79 . b Synthesis of labile benzo[ f ]oxazepines 85 . c Observations during attempted enzymatic conversion. Full size image Unfortunately, ester surrogates 79 proved unstable under the assay conditions, with even the enzyme-free negative control showing decomposition (Fig. 9c ). On the other hand, compounds 85 (freshly prepared) were observed to be reasonably stable in this environment, but no difference between negative control and AsqJ assay was observed. This may be a result of impurities contained in the crude substrate mixture that had to be employed due to the instability of 85 (see above), which might have inhibitory effects on AsqJ, or, more likely, be a consequence of the altered electronic and geometric properties of the ester vs . the natural amide substrates. Overall, these experiments lead to the conclusion that the central benzo[1,4]diazepine-2,5-dione motif is a required general precondition for AsqJ substrates. Quantification of the transformation of key substrates To investigate and compare AsqJ substrate preferences of the established and the newly discovered reactivities, we performed HPLC-based monitoring of substrate consumptions. We selected one representative substrate with high conversion for each of the described reaction trajectories towards different product classes. We hence utilized substrates 9c (quinazolin(di)one pathway), 10c (quinolone pathway), 49n (hydroxylation reactivity) and 54 (tricyclic substrate following quinazolinone pathway) for tracking of time-dependent substrate consumption by AsqJ. For each of these substrates, HPLC-UV concentration calibration curves at 220 nm were recorded and used to analyse substrate consumption in individual assays after 15, 60, 180 and 360 minutes (cf. ESI, chapter 3.4). This revealed that natural phenylalanine-derived substrate 10c was converted very fast, with 50% consumption after less than 40 minutes and more than 95% after 180 minutes. Hydroxylation of dimethylated glycine-derivative 49n and quinazolin(di)one formation from leucine-derived 9c were slower (50% consumption after approx. 100 and 120 minutes, respectively). However, after 360 minutes, conversion of approx. 90% was detected for both substrates. For proline-derived tricyclic 54 , conversion was generally slower and overall substrate consumption only reached 46% after 360 minutes. 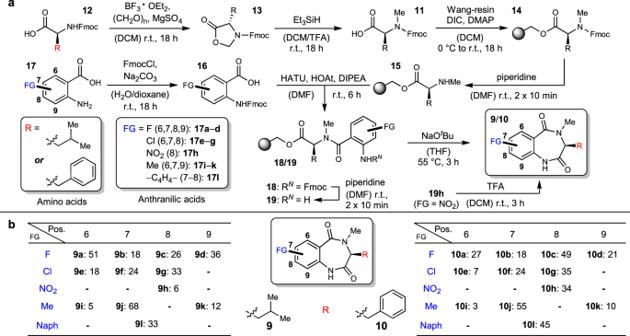Fig. 2: Combinatorial substrate synthesis by SPPS. aSynthetic route towardsN4-methylated benzo[1,4]diazepine-2,5-diones with different substitutions at the aromatic core, as indicated in blue.bOverall yields of the respective products9/10from14(over four steps). DCM dichloromethane, DICN,N’-diisopropylcarbodiimide, DIPEAN,N-diisopropylethylamine, DMAP 4-dimethylaminopyridine, DMFN,N-dimethylformamide, FG functional group, Fmoc fluorenylmethyloxycarbonyl, HATU hexafluorophosphate azabenzotriazole tetramethyl uronium, HOAt 1-hydroxy-7-azabenzotriazole, TFA trifluoroacetic acid, THF tetrahydrofuran. Overall, these investigations unsurprisingly revealed that AsqJ is most competent for transformation of its original, natural precursor structures such as 10c , but that catalytic efficiency also remains very high (for 9c, 49n ) to sufficient ( 54 ) for its biocatalytic application across all four investigated transformations (Fig. 10 ). Fig. 10: Substrate and product map of AsqJ. Overview over compounds/compound classes accessible by enzymatic conversion with AsqJ, as extended (red) and discovered (green) within this study. (Proposed) single reaction types are given with the reaction arrows. Full size image Within this work, we systematically evaluated the substrate promiscuity and product spectrum of the fungal dioxygenase AsqJ. While the experiments confirmed mechanistic proposals for the pathways representing the established bimodal activity of AsqJ, only quinolone formation turned out to be highly flexible, while quinazolinone formation was proven to have a rather narrow scope concerning the tested structural alterations of the substrate. The central seven-membered diamide structure was shown to be a necessary precondition for both, AsqJ enzymatic conversion and substrate stability. Moreover, by our broad-spectrum (cf. Table S1 ) substrate testing, we herein discovered the capability of AsqJ to generate tricyclic quinazolinones from tricyclic benzo[1,4]diazepine-2,5-diones, which can be applied in the synthesis of natural products, such as vasicinone ( 65 ). This is a highly interesting example of an enzyme that can be utilized to build a bridge between the biosynthesis of secondary metabolites of different kingdoms, as directly exemplified by the AsqJ-catalysed formation of deoxyvasicinone ( 64 ), isovasicinone ( 66 ) and mackinazolinone ( 72 ). Most importantly, our in-depth studies moreover revealed another heterocyclic compound class accessible by AsqJ, namely quinazolin-2,5-diones 22 / 44 . Mechanistic studies involving a 13 C-isotope labelled substrate 23 revealed this product class to be formed simultaneous to the corresponding quinazolinones and led us to the assumption that the side chain is oxidatively excised from the starting material (see Fig. S61 for a mechanistic proposal). Additionally, the biocatalytic formation of hydroxylated compounds such as 50 from unsubstituted (with respect to R 1 , Fig. 1e ) substrates opens the door for further studies towards the application of AsqJ for the synthesis of bioactive diazepines (as indicated by the structural similarity of 50 to lorazepam ( 51 )). Taken together, the extensive substrate promiscuity and resulting product diversity (cf. Table S2 ), as uncovered within this study, highlight a remarkable substrate-controlled product selectivity switch in the fascinating dioxygenase AsqJ. This work thus establishes AsqJ as a highly variable and sustainable tool for the generation of a whole set of bioactive compounds with diverse heterocyclic core structures by only subtle structural changes of the employed substrates (Fig. 10 ). Overall, our work has comprehensively mapped the substrate scope across the two previously known AsqJ reaction pathways and has resulted in the discovery of the biocatalytic competence of AsqJ to transform tricyclic substrates in addition to establishing two additional reactivities: side-chain excision to quinazolin-2,5-diones and substrate C 3 -hydroxylation. Further work towards the optimization of reaction conditions to enable large-scale preparative application of AsqJ is currently ongoing in our laboratories. General procedure of analytical enzyme assay Analytical enzymatic assays were carried out in a total volume of 120–350 µL, containing 1 m m of the substrate (dissolved in DMF: 100 m m ), 50 µm (5 mol-%) of purified AsqJ, 2.5 m m α-ketoglutarate, 4 m m ascorbic acid, 100 µ m iron(II) sulphate and 5% (v/v) DMF. 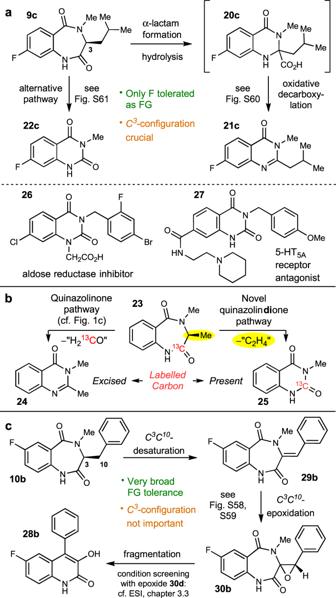Fig. 3: AsqJ assay results for selected substrates. aSummary of substrate screening outcomes for the quinazolin(di)one pathway (exemplarily shown for9c) and structures of quinazolindione biomedical agents26and27.bDifference in ring contraction for quinazolinone and quinazolindione products as observed by conversion of13C-labelled substrate23.cSummary of substrate screening outcomes for the quinolone pathway (exemplarily shown for10b). HT hydroxytryptamine. The reaction buffer contained 50 mm TRIS HCl at a pH of 7.4. 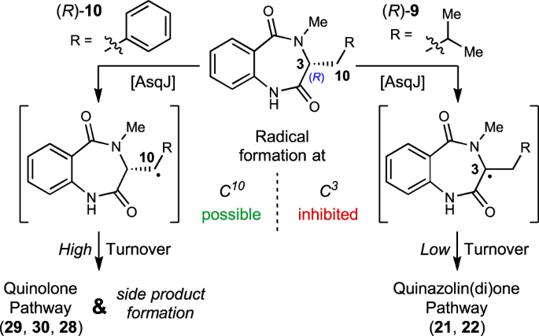Fig. 4: Investigations of substrate stereochemical influence. Results of enzyme assays with (R)-enantiomers of9and10and supposed explanation. After incubation for 5–6 h (8 h max.) with shaking at 300 rpm, the enzyme was precipitated by addition of TFA (1 µL TFA/40 µL assay) and removed by centrifugation for 5 min at 9700 × g . The supernatant (20 µL) was analysed by HPLC (Knauer Azura) at 220 nm with coupled ESI-MS (Advion, single-quadrupole mass analyser). 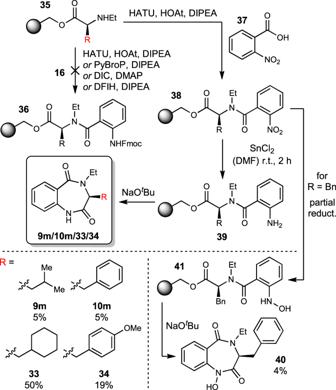Fig. 5: Optimized synthesis ofN4-ethylated substrates18. Yields are given over seven steps, starting from loaded resin. DFIH 1,3-dimethyl-2-fluoro-4,5-dihydro-1H-imidazolium hexafluorophosphate, PyBroP bromotripyrrolidinophosphonium hexafluorophosphate. 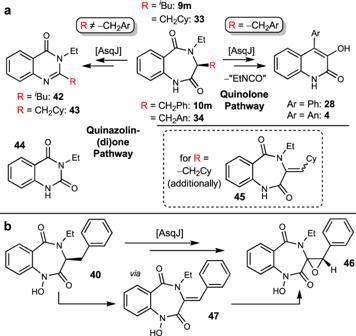Fig. 6: AsqJ assay results withN4-ethyl analogues. aBiocatalytic transformation ofN4-ethylated substrates.bConversion of the additionallyN1-hydroxylated analogue40, where no quinolone formation was observed. Cy cyclohexyl, An 4-anisolyl (p-methoxyphenyl). 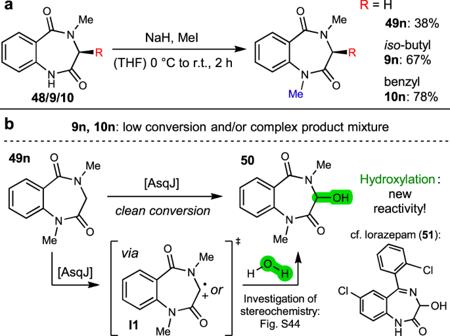Fig. 7: Synthesis and conversion ofN,N-dimethylated substrates. aLate-stage methylation (blue) towards the desired compounds.bResults of enzymatic conversion with mechanism proposal for hydroxylation of49n(proposed origin of hydroxyl group labelled in green), as well as structure of blockbuster pharmaceutical lorazepam (51). 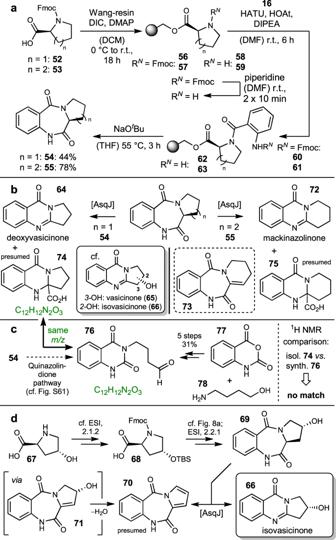Fig. 8: Investigations involving tricyclic substrates. aSynthesis of tricyclic substrates54/55.bEnzymatic conversion.cSynthesis of hypothesized aldehyde76and comparison with isolated compound74. Green colour indicates same chemical formulas and hencem/zratios of these compounds.dSynthesis and conversion ofl-4-hydroxyproline-derived substrate69. NMR nuclear magnetic resonance, TBStert-butyldimethylsilyl. 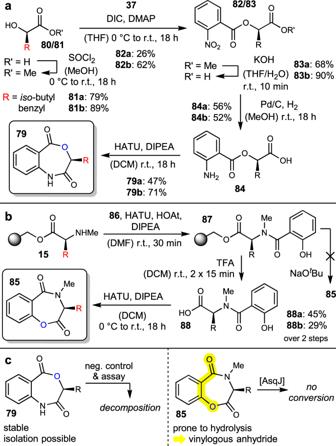Fig. 9: Syntheses and assays of ester substrate analogues. aRoute to benzo[e]oxazepines79.bSynthesis of labile benzo[f]oxazepines85.cObservations during attempted enzymatic conversion. 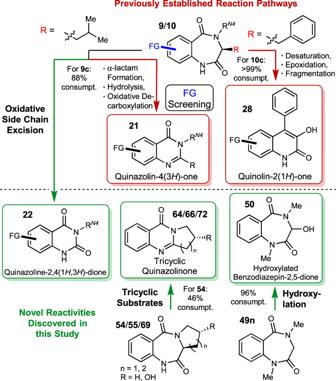Fig. 10: Substrate and product map of AsqJ. Overview over compounds/compound classes accessible by enzymatic conversion with AsqJ, as extended (red) and discovered (green) within this study. (Proposed) single reaction types are given with the reaction arrows. Experimental details and data Experimental procedures, like enzyme expression and purification, synthetic details, enzyme transformations for structure elucidation, as well as analytical characterization of compounds, comprising chromatograms, UV and NMR spectra are provided in the supplementary information.